SNAP-25 regulates spine formation through postsynaptic binding to p140Cap Synaptosomal-associated protein of 25 kDa (SNAP-25) is a member of the Soluble N -ethylmaleimide-sensitive-factor attachment protein receptors (SNARE) protein family, required for exocytosis of synaptic vesicles and regulation of diverse ion channels. Here, we show that acute reduction of SNAP-25 expression leads to an immature phenotype of dendritic spines that are, consistently, less functional. Conversely, over-expression of SNAP-25 results in an increase in the density of mature, Postsynaptic Density protein 95 (PSD-95)-positive spines. The regulation of spine morphogenesis by SNAP-25 depends on the protein’s ability to bind both the plasma membrane and the adaptor protein p140Cap, a key protein regulating actin cytoskeleton and spine formation. We propose that SNAP-25 allows the organization of the molecular apparatus needed for spine formation by recruiting and stabilizing p140Cap. Synaptosomal-associated protein of 25 kDa (SNAP-25) is a member of the SNARE protein family that comprises synaptobrevin/Vesicle-associated membrane protein (VAMP), syntaxin and SNAP-25, which are essential for the exocytosis of synaptic vesicles [1] , [2] , [3] . SNAP-25 is associated to cell membranes through palmitoylated cysteines that are located at the center of the protein [4] , [5] . SNAP-25 not only regulates exocytosis, but also negatively modulates different ion channels, including voltage-gated calcium channels (VGCCs) of N-type, P/Q-type and L-type [6] . Although SNAP-25 has a crucial role at the presynaptic level, a possible postsynaptic role of the protein has been proposed in the regulation of N -methyl- D -aspartate (NMDA) and kainate receptor (KAR) trafficking [7] , [8] . SNAP-25 has also been demonstrated to bind to p140Cap [9] , a 140-kDa protein mainly present in brain, testis and epithelial-rich tissues. In breast cancer cells, p140Cap negatively regulates cell spreading, motility, growth [10] and invasion [11] , affecting tumour cell properties. In neurons, p140Cap is localized in both the pre- and post-synaptic compartments [12] , [13] and its silencing leads to a decrease in the number of mature mushroom spines, thus providing evidence that p140Cap has a key role in the control of synaptic remodelling. Rearrangements of the actin cytoskeleton are believed to be of fundamental importance for changes in the morphology of dendritic spines [14] , [15] . Interestingly, spine formation and maintenance have been recently found to be controlled by genes involved in energy metabolism [16] . Spines can vary significantly in size and shape, from long filopodial spines to stubby and mushroom mature spines [17] , [18] . Several evidences correlate the size of the spine with the strength of the synapse, hinting at a possible structural mechanism at the basis of learning and memory [19] , [20] , [21] . Consistently, abnormal spine morphology and density has been described in a number of psychiatric diseases [18] , [22] , [23] , thus clearly indicating that proteins regulating spine remodelling and dynamics are fundamental molecular players in different pathologies of the nervous system. The SNAP-25 gene has been associated to different neuropsychiatric diseases, including schizophrenia, attention deficit hyperactivity disorder and bipolar disorder [24] , [25] , [26] , [27] , and defective SNAP-25 function has been shown to be responsible for neurodegeneration in cysteine-string protein (CSP)-alpha KO mice [28] . We therefore investigated whether SNAP-25 may have a role in the regulation of spine morphology through its binding to p140Cap. We demonstrate that SNAP-25 can recruit p140Cap and regulate density, morphology and functionality of dendritic spines. These data unveil an unexpected key role of SNAP-25 in the morphogenesis of the postsynaptic compartment. SNAP-25 regulates dendritic spine density and function We have previously shown that transfection of rat hippocampal neurons with a pSuper vector containing nucleotides 321–339 of rat SNAP-25 reduces SNAP-25 expression by ~60% at 1–2 days after transfection [29] , [30] . Acute downregulation of SNAP-25 by siRNA resulted in an unexpected morphological dendrite alteration. 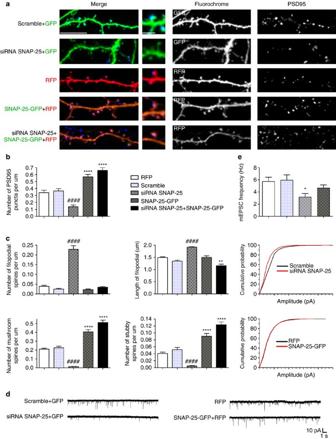Figure 1: Effect of SNAP-25 silencing or over-expression on spine morphology and function. (a) PSD-95 immunocytochemical staining of 20 DIV old rat hippocampal cultures silenced for SNAP-25 and transfected with GFP; transfected with SNAP-25-GFP and RFP; and silenced for SNAP-25 (rat construct) and transfected for SNAP-25-GFP (mouse construct) and RFP; Scale bar 10 μm (scale bar inset 2.5 μm). (b) Quantitative analysis of PSD95 immunoreactivity. Scramble:n=4 independent experiments, neurons=49, siRNA SNAP-25:n=3, neurons=47, RFP:n=6, neurons=45, SNAP-25:n=3, neurons=34, siRNA SNAP-25+SNAP-25n=3, neurons=40. Values are mean±s.e.m. Statistical test: **** and####P≤0.0001; one-way ANOVA was followed by Bonferroni multiple-comparisonpost hoctests. (c) Quantitative analysis of spine density and filopodial length. Scramble:n=4 independent experiments, neurons=46, siRNA SNAP-25:n=3, neurons=60, RFP:n=9, neurons=85, SNAP-25:n=5, neurons=51, siRNA SNAP-25+SNAP-25n=3, neurons=40. Values are mean±s.e.m. Statistical test: **** or####P≤0.0001, **P≤0.01; one-way ANOVA followed by Bonferroni multiple-comparisonpost hoctests. (d) Representative traces of mEPSC recordings in neurons silenced for SNAP-25 or transfected with SNAP-25-GFP. (e) Top panel: mEPSC frequency. Scramble:n=4 independent experiments, neurons=13, siRNA SNAP-25:n=4, neurons=11,P≤0.05; RFP:n=4, neurons=11 versus SNAP-25:n=4, neurons=12. Values are mean±s.e.m. *P≤0.05; statistical test: Mann-Whitneyt-test. Middle and bottom panels: cumulative distribution of mEPSC amplitude (scramble:n=4 independent experiments, neurons=13 versus siRNA SNAP-25:n=4, neurons=11,P≤0.05; RFP:n=4, neurons=11 versus SNAP-25n=4, neurons=12, ns. Statistical test: Two-sample Kolmogorov–Smirnov test). Figure 1a–c shows the quantitative analysis of 20 days in vitro (DIV) primary rat hippocampal cultures, co-transfected at 17 DIV with SNAP-25 siRNA and green fluorescent protein (GFP), and stained for the postsynaptic marker PSD95. A significant decrease in the number of mushroom and stubby spines could be detected upon the reduction of SNAP-25 expression. Conversely, a strong increase in the number of filopodia was observed ( Fig. 1a and c ). The decrease in the number of mature spines in the silenced neurons was mirrored by the reduced density of PSD95 ( Fig. 1a ), while over-expression of SNAP-25-GFP (ref. 29 ) in 17 DIV hippocampal neurons resulted in an increase in the number of mature spines and of PSD95 puncta ( Fig. 1a–c ), further indicating a role for SNAP-25 in the maturation of dendritic spines in primary cultures. To evaluate whether the decrease in mature spines in the absence of SNAP-25 could be rescued by protein re-expression, mouse SNAP-25-GFP, which is not knocked down by the rat siRNA construct, was transfected in hippocampal neurons in which endogenous SNAP-25 was simultaneously silenced. Over-expression of SNAP-25 in these cells led to the rescue of the silenced phenotype by decreasing the number of filopodial spines and increasing the number of mushroom and stubby spines as well as of PSD95 puncta ( Fig. 1a–c ). Figure 1: Effect of SNAP-25 silencing or over-expression on spine morphology and function. ( a ) PSD-95 immunocytochemical staining of 20 DIV old rat hippocampal cultures silenced for SNAP-25 and transfected with GFP; transfected with SNAP-25-GFP and RFP; and silenced for SNAP-25 (rat construct) and transfected for SNAP-25-GFP (mouse construct) and RFP; Scale bar 10 μm (scale bar inset 2.5 μm). ( b ) Quantitative analysis of PSD95 immunoreactivity. Scramble: n =4 independent experiments, neurons=49, siRNA SNAP-25: n =3, neurons=47, RFP: n =6, neurons=45, SNAP-25: n =3, neurons=34, siRNA SNAP-25+SNAP-25 n =3, neurons=40. Values are mean±s.e.m. Statistical test: **** and #### P ≤0.0001; one-way ANOVA was followed by Bonferroni multiple-comparison post hoc tests. ( c ) Quantitative analysis of spine density and filopodial length. Scramble: n =4 independent experiments, neurons=46, siRNA SNAP-25: n =3, neurons=60, RFP: n =9, neurons=85, SNAP-25: n =5, neurons=51, siRNA SNAP-25+SNAP-25 n =3, neurons=40. Values are mean±s.e.m. Statistical test: **** or #### P ≤0.0001, ** P ≤0.01; one-way ANOVA followed by Bonferroni multiple-comparison post hoc tests. ( d ) Representative traces of mEPSC recordings in neurons silenced for SNAP-25 or transfected with SNAP-25-GFP. ( e ) Top panel: mEPSC frequency. Scramble: n =4 independent experiments, neurons=13, siRNA SNAP-25: n =4, neurons=11, P ≤0.05; RFP: n =4, neurons=11 versus SNAP-25: n =4, neurons=12. Values are mean±s.e.m. * P ≤0.05; statistical test: Mann-Whitney t -test. Middle and bottom panels: cumulative distribution of mEPSC amplitude (scramble: n =4 independent experiments, neurons=13 versus siRNA SNAP-25: n =4, neurons=11, P ≤0.05; RFP: n =4, neurons=11 versus SNAP-25 n =4, neurons=12, ns. Statistical test: Two-sample Kolmogorov–Smirnov test). Full size image Electrophysiological analysis of SNAP-25 silenced cultures revealed that both the frequency and the amplitude of miniature excitatory postsynaptic currents (mEPSCs) were significantly reduced ( Fig. 1d ). Conversely, over-expression of SNAP-25 did not lead to increase of mEPCS frequency or amplitude ( Fig. 1d ). SNAP-25 membrane binding is required for spine formation It has been previously shown that SNAP-25, acting as a SNARE in the postsynaptic compartment, regulates the insertion and removal of postsynaptic NMDA and KARs [7] , [8] . We therefore reasoned that SNAP-25 could contribute to spine formation by mediating the insertion of postsynaptic components into the dendritic membrane. To directly test this possibility, we took advantage of the C-terminal deletion mutants SNAP-25Δ 198–206 , the fragment generated by botulinum neurotoxin/A (BoNT/A) action, or SNAP-25Δ 181–206 , the fragment generated by botulinum neurotoxin/E (BoNT/E) action, that do not sustain exocytosis [31] , [32] ( Fig. 2a ). Both constructs, fused to HA, were visualized by double immunofluorescence with a FITC-secondary antibody. Over-expression of either SNAP-25Δ 181–206 or SNAP-25Δ 198–206 led to a phenotype similar to that induced by full-length SNAP-25, that is, increase in stubby and mushroom spines ( Fig. 2b ). To exclude that endogenous SNAP-25 could contribute a SNARE function, co-transfection of SNAP-25Δ 198–206 in cells silenced for SNAP-25 was carried out, resulting again in an increase in stubby and mushroom spines compared to control neurons ( Fig. 2b ). Conversely, over-expression of the SNAP-25 mutant SNAP-25Δ 86–120 ( Fig. 2a ), which is devoid of the inter-helical domain of the protein controlling its localization at the plasma membrane [5] (see also Supplementary Fig. S1 ), produced an increase in the number of filopodial spines and decrease in stubby and mushroom protrusions ( Fig. 2b ). Therefore, the effect of SNAP-25 on spine morphology relies on its ability to bind to the plasma membrane. 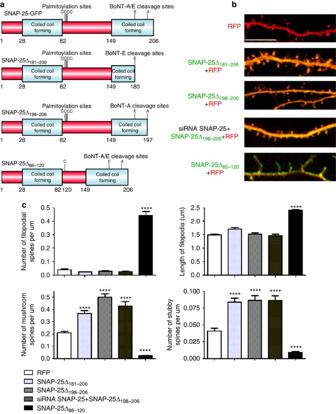Figure 2: SNAP-25 binding to the membrane is required for its effect on spine morphology. (a) Schematic representation of the constructs used in these experiments (SNAP-25Δ198–206and SNAP-25Δ181–206, lacking the SNARE function and SNAP-25Δ86–120lacking the ability to interact with the plasma membrane). (b) Immunocytochemical staining of 20 DIV rat hippocampal neurons transfected with RFP or co-transfected with SNAP-25Δ198–206or with SNAP-25Δ181–206fused to a HA tag (subsequently labelled for HA) and RFP or with SNAP-25Δ86–120fused to GFP and RFP. Scale bar 10 μm. (c) Quantitative analysis of filopodial, stubby and mushroom spine density and of filopodial spines length in 20 DIV rat hippocampal neurons transfected as above. RFP:n=9 independent experiments, neurons=85; SNAP-25Δ181–206:n=3 independent experiments, neurons=41; SNAP-25Δ198–206:n=3 independent experiments, neurons=42; siRNA SNAP-25+SNAP-25Δ198–206:n=3 independent experiments, neurons=27; SNAP-25Δ86–120:n=3 independent experiments, neurons=41. Values are mean±s.e.m. Statistical test: ****P≤0.0001; one-way ANOVA followed by Bonferroni multiple-comparisonpost hoctests. Figure 2: SNAP-25 binding to the membrane is required for its effect on spine morphology. ( a ) Schematic representation of the constructs used in these experiments (SNAP-25Δ 198–206 and SNAP-25Δ 181–206 , lacking the SNARE function and SNAP-25Δ 86–120 lacking the ability to interact with the plasma membrane). ( b ) Immunocytochemical staining of 20 DIV rat hippocampal neurons transfected with RFP or co-transfected with SNAP-25Δ 198–206 or with SNAP-25Δ 181–206 fused to a HA tag (subsequently labelled for HA) and RFP or with SNAP-25Δ 86–120 fused to GFP and RFP. Scale bar 10 μm. ( c ) Quantitative analysis of filopodial, stubby and mushroom spine density and of filopodial spines length in 20 DIV rat hippocampal neurons transfected as above. RFP: n =9 independent experiments, neurons=85; SNAP-25Δ 181–206 : n =3 independent experiments, neurons=41; SNAP-25Δ 198–206 : n =3 independent experiments, neurons=42; siRNA SNAP-25+SNAP-25Δ 198–206 : n =3 independent experiments, neurons=27; SNAP-25Δ 86–120 : n =3 independent experiments, neurons=41. Values are mean±s.e.m. Statistical test: **** P ≤0.0001; one-way ANOVA followed by Bonferroni multiple-comparison post hoc tests. Full size image p140Cap regulates spine density and function Given the SNARE function of the protein does not seem to be required for spine morphogenesis, we hypothesized that SNAP-25 may be required as a scaffolding protein to control the plasma membrane localization of protein complexes controlling spine formation. Among these proteins, p140Cap, which localizes to synapses and is required for spine maintenance [12] , [13] , [33] , is known to interact with SNAP-25 [9] . Consistently, SNAP-25 and p140Cap co-immunoprecipitated upon transfection in Human Embryonic Kidney-293 (HEK-293) cells ( Supplementary Fig. S2 ); on the other hand, co-transfection of p140Cap and SNAP-25Δ 1–41 , a SNAP-25 mutant construct lacking the N-terminal region required for binding to p140Cap [9] , resulted in ~85% reduction of co-immunoprecipitation ( Supplementary Fig. S2 ). When overexpressed in neuronal cultures, SNAP-25-GFP, similarly to p140Cap-GFP, was partially detectable in dendritic spines ( Supplementary Fig. S3a ). To investigate the possible endogenous localization of the protein in the dendritic compartment ( Supplementary Fig. S3b ), we used the IMARIS reconstruction ( Supplementary Fig. S3c ) or ground state depletion (GSD) technique ( Supplementary Fig. S3d ), focusing on neuronal regions receiving low axonal inputs, where SNAP-25 is predominantly localized [34] . Consistently, and differently from presynaptic proteins such as synaptophysin and the calcium subunit alpha 1a/CaV2.1 (ref. 35 ), SNAP-25 was also detected, together with p140Cap and a small amount of the SNARE Syntaxin1, in a highly purified post-synaptic density fraction (PSD) from adult rat hippocampus ( Supplementary Fig. S3e ) [36] . Staining of hippocampal neurons with SNAP-25 and p140Cap showed that the two proteins are sporadically detectable at the level of the same dendritic protrusion ( Supplementary Fig. S3f ). Consistently, and in line with the known interaction between SNAP-25 and p140Cap (ref. 9 ), coimmunoprecipitation experiments in rodent brain revealed that p140Cap and SNAP-25 are part of the same molecular complex, which also comprises PSD-95 ( Supplementary Fig. S3g ). Transfection of DIV 17 rat hippocampal neurons with a cDNA coding mouse p140Cap-GFP (bearing GFP at the C-terminal) [10] , or a cDNA coding mouse p140Cap-NterGFP (bearing GFP at the N-terminal) [13] or with pSuper Retro-p140 encoding for specific rat p140Cap shRNA [37] confirmed previous results [13] : similarly to SNAP-25, p140Cap silencing led to a decrease in the number of stubby and mushroom spines and of PSD95 puncta [13] ( Fig. 3a–c ), while over-expression of the protein led to an increase of stubby and mushroom spines ( Fig. 3a and Supplementary Fig. S4 ), as well as of PSD95 puncta ( Fig. 3a ). As a control, over-expression of human p140Cap, which is not knocked down by the rat shRNA, in neurons silenced for the endogenous protein, led to the rescue of the spine phenotype ( Fig. 3a–c ). Electrophysiological recording showed that p140Cap knockdown recordings reduced mEPSCs frequency but had no effect on mEPSCs amplitude ( Fig. 3d ). Similarly to SNAP-25, p140Cap over-expression did not result in significant changes in either amplitude or frequency of mEPSCs ( Fig. 3d ). 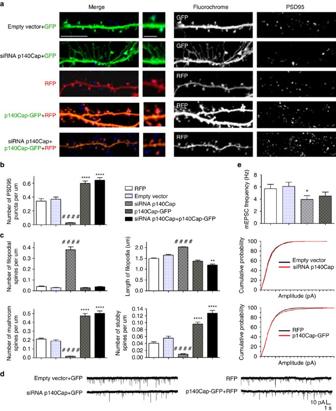Figure 3: Effect of p140Cap silencing and over-expression on spine morphology and function. (a) PSD-95 immunocytochemical staining of 20 DIV-old rat hippocampal cultures silenced for p140Cap and transfected with GFP; transfected with p140-GFP and RFP; and silenced for rat p140 and transfected with human p140Cap-GFP and RFP; scale bar: 10 μm (scale bar insert: 2.5 μm). (b) Quantitative analysis of PSD95 puncta in 20 DIV neurons. Empty vector:n=3 independent experiments, neurons=30; siRNA p140Cap:n=3, neurons=45; RFP:n=6, neurons=45; p140Cap-GFP:n=3, neurons=32; siRNA p140Cap+p140Cap n=3, neurons=41. Values are mean±s.e.m. Statistical test: **** and####P≤0.0001; one-way ANOVA followed by Bonferroni multiple-comparisonpost hoctests. (c) Quantitative analysis of spine density and of filopodial spine length. Empty vector:n=4 independent experiments, neurons=40; siRNA p140Cap:n=5, neurons=75; RFP:n=9, neurons=85; p140Cap:n=4, neurons=42; siRNA p140Cap+p140Cap:n=4, neurons=41. Values are mean±s.e.m. Statistical test: **** and####P≤0.0001, **P≤0.01; one-way ANOVA followed by Bonferroni multiple-comparisonpost hoctests. (d) Representative traces of mEPSC recordings from 20 DIV rat hippocampal neurons silenced for p140Cap or transfected with p140Cap. (e) Top panel: average mEPSC frequency. Empty:n=4 independent experiments, neurons=10, siRNA p140Cap:n=4, neurons=10, RFP:n=4, neurons=11; p140Cap:n=4, neurons=15. Values are mean±s.e.m. *P≤0.05 Statistical test: Mann–Whitneyt-test. Middle and bottom panels: cumulative distribution of mEPSC amplitude (empty:n=4 independent experiments, neurons=10 versus siRNA p140Cap:n=4, neurons=10, ns. RFP:n=4, neurons=11 versus p140Cap:n=4, neurons=15, ns. Statistical test: Two-sample Kolmogorov–Smirnov test.). Figure 3: Effect of p140Cap silencing and over-expression on spine morphology and function. ( a ) PSD-95 immunocytochemical staining of 20 DIV-old rat hippocampal cultures silenced for p140Cap and transfected with GFP; transfected with p140-GFP and RFP; and silenced for rat p140 and transfected with human p140Cap-GFP and RFP; scale bar: 10 μm (scale bar insert: 2.5 μm). ( b ) Quantitative analysis of PSD95 puncta in 20 DIV neurons. Empty vector: n =3 independent experiments, neurons=30; siRNA p140Cap: n =3, neurons=45; RFP: n =6, neurons=45; p140Cap-GFP: n =3, neurons=32; siRNA p140Cap+p140Cap n=3, neurons=41. Values are mean±s.e.m. Statistical test: **** and #### P ≤0.0001; one-way ANOVA followed by Bonferroni multiple-comparison post hoc tests. ( c ) Quantitative analysis of spine density and of filopodial spine length. Empty vector: n =4 independent experiments, neurons=40; siRNA p140Cap: n =5, neurons=75; RFP: n =9, neurons=85; p140Cap: n =4, neurons=42; siRNA p140Cap+p140Cap: n =4, neurons=41. Values are mean±s.e.m. Statistical test: **** and #### P ≤0.0001, ** P ≤0.01; one-way ANOVA followed by Bonferroni multiple-comparison post hoc tests. ( d ) Representative traces of mEPSC recordings from 20 DIV rat hippocampal neurons silenced for p140Cap or transfected with p140Cap. ( e ) Top panel: average mEPSC frequency. Empty: n =4 independent experiments, neurons=10, siRNA p140Cap: n =4, neurons=10, RFP: n =4, neurons=11; p140Cap: n =4, neurons=15. Values are mean±s.e.m. * P ≤0.05 Statistical test: Mann–Whitney t -test. Middle and bottom panels: cumulative distribution of mEPSC amplitude (empty: n =4 independent experiments, neurons=10 versus siRNA p140Cap: n =4, neurons=10, ns. RFP: n =4, neurons=11 versus p140Cap: n =4, neurons=15, ns. Statistical test: Two-sample Kolmogorov–Smirnov test.). Full size image Spine remodelling requires SNAP-25 and p140Cap association Over-expression of p140Cap in cells silenced for SNAP-25 ( Fig. 4 ) or over-expression of SNAP-25 in cells silenced for p140Cap ( Fig. 5 ) led to an immature spine phenotype, characterized by increased filopodial spines number and a decrease in mushroom and stubby spine numbers ( Fig. 5 ). These data suggest that SNAP-25 and p140Cap are both necessary for the regulation of dendritic spine morphology, possibly through protein–protein interactions. 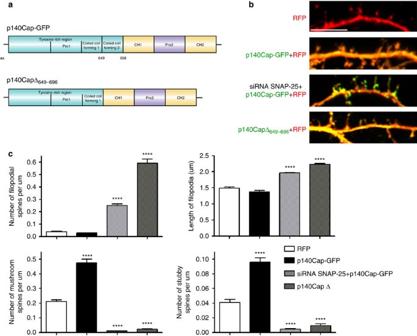Figure 4: p140Cap needs SNAP-25 to affect spine morphology. (a) Schematic representation of the constructs used in these experiments (p140CapΔ649–696lacking the region necessary for interaction with SNAP-25). (b) Immunocytochemistry of 20 DIV rat hippocampal neurons transfected with RFP or co-transfected with RFP and p140Cap-GFP, with RFP and p140Cap-GFP and silenced for SNAP-25 or with RFP and p140CapΔ649–696. Scale bar: 10 μm. (c) Quantitative analysis of filopodial, stubby and mushroom spine density and of filopodial spine length in 20 DIV rat hippocampal neurons. RFP:n=9 independent experiments, neurons=85; siRNA SNAP-25+p140Cap:n=3 independent experiments, neurons=41; p140CapΔ649–696:n=3 independent experiments, neurons=30. Values are mean±s.e.m. Statistical test: ****P≤0.0001; one-way ANOVA followed by Bonferroni multiple-comparisonpost hoctests. Figure 4: p140Cap needs SNAP-25 to affect spine morphology. ( a ) Schematic representation of the constructs used in these experiments (p140CapΔ 649–696 lacking the region necessary for interaction with SNAP-25). ( b ) Immunocytochemistry of 20 DIV rat hippocampal neurons transfected with RFP or co-transfected with RFP and p140Cap-GFP, with RFP and p140Cap-GFP and silenced for SNAP-25 or with RFP and p140CapΔ 649–696 . Scale bar: 10 μm. ( c ) Quantitative analysis of filopodial, stubby and mushroom spine density and of filopodial spine length in 20 DIV rat hippocampal neurons. RFP: n =9 independent experiments, neurons=85; siRNA SNAP-25+p140Cap: n =3 independent experiments, neurons=41; p140CapΔ 649–696 : n =3 independent experiments, neurons=30. Values are mean±s.e.m. Statistical test: **** P ≤0.0001; one-way ANOVA followed by Bonferroni multiple-comparison post hoc tests. 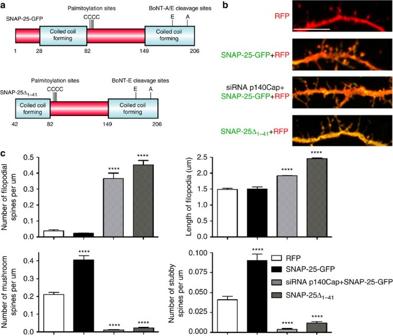Figure 5: SNAP-25 needs p140Cap to affect spine morphology. (a) Schematic representation of the constructs used in these experiments (SNAP-25Δ1–41lacking the region required for interaction with p140Cap). (b) Immunocytochemistry of 20 DIV rat hippocampal neurons transfected with RFP or co-transfected with RFP and SNAP-25-GFP, with RFP and SNAP-25-GFP and silenced for p140Cap or with RFP and SNAP-25Δ1–41. Scale bar 10 μm. (c) Quantitative analysis of filopodial, stubby and mushroom spine density and of filopodial spine length in 20 DIV rat hippocampal neurons. RFP:n=9 independent experiments, neurons=85; siRNA p140Cap+SNAP-25:n=3 independent experiments, neurons=41; SNAP-25Δ1–41:n=4 independent experiments, neurons=53. Values are mean±s.e.m. Statistical test: ****P≤0.0001; one-way ANOVA followed by Bonferroni multiple-comparisonpost hoctests. Full size image Figure 5: SNAP-25 needs p140Cap to affect spine morphology. ( a ) Schematic representation of the constructs used in these experiments (SNAP-25Δ 1–41 lacking the region required for interaction with p140Cap). ( b ) Immunocytochemistry of 20 DIV rat hippocampal neurons transfected with RFP or co-transfected with RFP and SNAP-25-GFP, with RFP and SNAP-25-GFP and silenced for p140Cap or with RFP and SNAP-25Δ 1–41 . Scale bar 10 μm. ( c ) Quantitative analysis of filopodial, stubby and mushroom spine density and of filopodial spine length in 20 DIV rat hippocampal neurons. RFP: n =9 independent experiments, neurons=85; siRNA p140Cap+SNAP-25: n =3 independent experiments, neurons=41; SNAP-25Δ 1–41 : n =4 independent experiments, neurons=53. Values are mean±s.e.m. Statistical test: **** P ≤0.0001; one-way ANOVA followed by Bonferroni multiple-comparison post hoc tests. Full size image To univocally demonstrate this possibility, we transfected primary hippocampal neurons with a p140Cap construct deleted of amino acids (aa) 649–696, which are essential for binding to SNAP-25 (ref. 9 ) (p140CapΔ 649–696 ) ( Fig. 4a ). An increase in the number of filopodial spines and a decrease in the number of stubby and mushroom spines were observed after transfection with p140CapΔ 649–696 ( Fig. 4b ). Transfection of hippocampal neurons with SNAP-25Δ 1–41 ( Fig. 5a ), a SNAP-25 mutant construct lacking the N-terminal region required for binding to p140Cap (ref. 9 ), led to an increase in the number of filopodial spines and a decrease of stubby and mushroom spines ( Fig. 5b ). The inability of SNAP-25Δ 1–41 to bind p140Cap was demonstrated by co-immunoprecipitation assays in HEK-293 cells ( Supplementary Fig. S2 ). These results indicate that SNAP-25 and p140Cap need to associate in order to drive a cooperative regulation of spine morphology. p140Cap localization requires membrane binding of SNAP-25 To investigate whether SNAP-25 and p140Cap control their reciprocal localization, we carried out transfection of different constructs in Hela cells ( Supplementary Fig. S1 ). While SNAP-25-GFP over-expressed in Hela cells colocalized with subcortical actin fibres [38] ( Supplementary Fig. S1a , see also high magnification insert), SNAP-25Δ 86–120 , which lacks the region required for binding to the plasmamembrane, was clearly delocalized from the cell surface ( Supplementary Fig. S1b , see also high magnification insert). p140Cap-myc, visualized by staining with anti myc antibodies, was concentrated around the perinuclear, putative Golgi, area ( Supplementary Fig. S1c ). Notably, co-transfection of SNAP-25-GFP resulted in the delocalization of p140Cap-myc from the Golgi area, leading to a more diffuse distribution of the protein ( Supplementary Fig. S1d ). Conversely, co-transfection of p140Cap-myc and SNAP-25Δ 1–41 , which lacks the p140Cap interaction domain, did not lead to delocalization of p140Cap, which maintained instead its distribution around the nucleus ( Supplementary Fig. S1e ). Similar results were obtained upon co-transfection of SNAP-25 with p140Cap lacking the SNAP-25 interacting domain ( Supplementary Fig. S1f ). Quantitative analysis ( Supplementary Fig. S1g ) confirmed that, when coexpressed with SNAP-25 lacking either the plasmamembrane- or the p140Cap-interacting regions, p140Cap displayed a significantly lower colocalization with subcortical actin. Consistently, the p140 construct lacking the SNAP-25 interacting domain displayed a reduced colocalization with subcortical actin, even if coexpressed with wt SNAP-25 ( Supplementary Fig. S1g ). To investigate whether SNAP-25 controls the localization of p140Cap also in neuronal cells, the p140Cap-NterGFP ( Supplementary Fig. S4 ) was transfected with SNAP-25 scramble or siRNA-transfected neurons ( Fig. 6 ). Over-expression of p140Cap-NterGFP together with the SNAP-25 scramble pSuper vector construct showed the typical enrichment of p140Cap at the head of the dendritic spines [13] ( Fig. 6a ). Conversely, over-expression of p140Cap-NterGFP in SNAP-25-silenced neurons resulted in a different localization of p140Cap, which appeared diffuse and not concentrated at the tip of the protrusions ( Fig. 6b ). The reduction of p140Cap localization at dendritic spines in the absence of SNAP-25 was confirmed by a quantification of the intensity of p140Cap in spines versus the dendritic shaft ( Fig. 6c ). Similar results were obtained when assessing the impact of SNAP-25 downregulation on the localization of endogenous p140Cap ( Fig. 6d–f ). 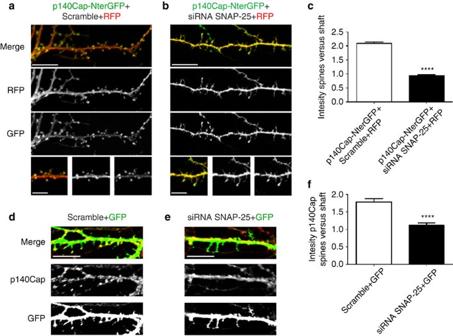Figure 6: SNAP-25 silencing delocalizes p140Cap. (a,b) Immunocytochemistry of 20 DIV rat hippocampal neurons co-transfected with RFP, p140Cap-NterGFP and scramble pSuper vector, or with RFP, p140Cap-NterGFP RFP and pSuper vector containing nucleotides 321–339 (siRNA) of rat SNAP-25. While p140Cap is enriched in dendritic spines of control neurons transfected with the scramble construct (a), neurons silenced for SNAP-25 show delocalization of p140Cap (b); Scale bar 10 μm, bottom 5 μm. (c) quantification of p140Cap-NterGFP spine targeting through the evaluation of fluorescence intensity in spines versus dendritic shafts of p140Cap-NterGFP in scramble or SNAP-25 siRNA-transfected neurons. p140Cap-NterGFP+scramble:n=3 independent experiments, neurons=30; p140Cap-NterGFP+siRNA SNAP-25:n=3 independent experiments, neurons=30. Values are mean±s.e.m. Statistical test: ****P≤0.0001; unpaired Student’st-test. (d,e) Immunocytochemistry of rat hippocampal neurons co-transfected with GFP and scramble pSuper vector, or with GFP and pSuper vector containing nucleotides 321–339 (siRNA) of rat SNAP-25. p140Cap is enriched in dendritic spines of control neurons (d), while in neurons silenced for SNAP-25, it is delocalized in the dendritic shaft (e). Scale bar: 10 μm. (f) Quantification of endogenous p140Cap through the evaluation of fluorescence intensity in spines versus dendritic shafts in scramble or SNAP-25 siRNA transfected neurons. Scramble:n=3 independent experiments, neurons=28, siRNA; SNAP-25: n=3 independent experiments, neurons=30. Values are mean±s.e.m. Statistical test: ****P≤0.0001; unpaired Student’st-test. Figure 6: SNAP-25 silencing delocalizes p140Cap. ( a , b ) Immunocytochemistry of 20 DIV rat hippocampal neurons co-transfected with RFP, p140Cap-NterGFP and scramble pSuper vector, or with RFP, p140Cap-NterGFP RFP and pSuper vector containing nucleotides 321–339 (siRNA) of rat SNAP-25. While p140Cap is enriched in dendritic spines of control neurons transfected with the scramble construct ( a ), neurons silenced for SNAP-25 show delocalization of p140Cap ( b ); Scale bar 10 μm, bottom 5 μm. ( c ) quantification of p140Cap-NterGFP spine targeting through the evaluation of fluorescence intensity in spines versus dendritic shafts of p140Cap-NterGFP in scramble or SNAP-25 siRNA-transfected neurons. p140Cap-NterGFP+scramble: n =3 independent experiments, neurons=30; p140Cap-NterGFP+siRNA SNAP-25: n =3 independent experiments, neurons=30. Values are mean±s.e.m. Statistical test: **** P ≤0.0001; unpaired Student’s t -test. ( d , e ) Immunocytochemistry of rat hippocampal neurons co-transfected with GFP and scramble pSuper vector, or with GFP and pSuper vector containing nucleotides 321–339 (siRNA) of rat SNAP-25. p140Cap is enriched in dendritic spines of control neurons ( d ), while in neurons silenced for SNAP-25, it is delocalized in the dendritic shaft ( e ). Scale bar: 10 μm. ( f ) Quantification of endogenous p140Cap through the evaluation of fluorescence intensity in spines versus dendritic shafts in scramble or SNAP-25 siRNA transfected neurons. Scramble: n =3 independent experiments, neurons=28, siRNA; SNAP-25: n=3 independent experiments, neurons=30. Values are mean±s.e.m. Statistical test: **** P ≤0.0001; unpaired Student’s t -test. Full size image To further prove SNAP-25 role in the localization of p140Cap, fluorescence recovery after photobleaching (FRAP) experiments were carried out ( Fig. 7a–c ). Neurons co-transfected with p140Cap-NterGFP and silenced for SNAP-25 showed a higher mobile fraction of p140Cap, compared to controls ( Fig. 7b ). The higher mobility of p140Cap in neurons lacking SNAP-25 was also confirmed by examining the recovery of fluorescence of p140Cap-NterGFP ( Fig. 7c ). Indeed, p140Cap fluorescence recovers in a greater extent when p140Cap-NterGFP is transfected in cells silenced for SNAP-25 compared to cells co-transfected with a scramble pSuper vector construct ( Fig. 7c ). These results indicate a role for SNAP-25 in the formation of mature spines by localizing p140Cap. 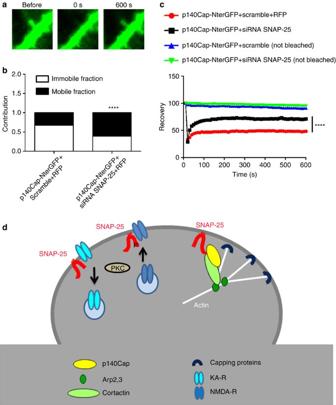Figure 7: SNAP-25 impacts p140Cap motility. (a) Examples of the fluorescence distribution and intensity of p140Cap-NterGFP before, directly after and 600 s after bleaching. (b) Average size of the mobile and immobile fractions of p140Cap-NterGFP measured by FRAP in neurons expressing SNAP-25 scramble or siRNA constructs. p140Cap-NterGFP+scramble:n=3 independent experiments, neurons=30, p140Cap-NterGFP+siRNA SNAP-25n=3 independent experiments, neurons=30. Values are mean. Statistical test: ****P≤0.0001 Statistical test: two-way ANOVA followed by Bonferroni multiple-comparisonpost hoctests. (c) Averaged time traces of fluorescence recovery after photobleaching for p140Cap-NterGFP in neurons transfected with scramble or SNAP-25 siRNA. Statistical test: two-way ANOVA. (d) The scheme depicts the mechanisms by which SNAP-25 contributes to postsynaptic function. SNAP-25 has a role in the removal of KARs8and in the insertion of NMDA receptors in neuronal plasma membrane7, both processes involving PKC. Furthermore, through the interaction with p140Cap, SNAP-25 may stabilize a postsynaptic complex including cortactin13, Arp2,3, actin and actin capping proteins51,60, thus having a role in spine morphogenesis. Figure 7: SNAP-25 impacts p140Cap motility. ( a ) Examples of the fluorescence distribution and intensity of p140Cap-NterGFP before, directly after and 600 s after bleaching. ( b ) Average size of the mobile and immobile fractions of p140Cap-NterGFP measured by FRAP in neurons expressing SNAP-25 scramble or siRNA constructs. p140Cap-NterGFP+scramble: n =3 independent experiments, neurons=30, p140Cap-NterGFP+siRNA SNAP-25 n =3 independent experiments, neurons=30. Values are mean. Statistical test: **** P ≤0.0001 Statistical test: two-way ANOVA followed by Bonferroni multiple-comparison post hoc tests. ( c ) Averaged time traces of fluorescence recovery after photobleaching for p140Cap-NterGFP in neurons transfected with scramble or SNAP-25 siRNA. Statistical test: two-way ANOVA. ( d ) The scheme depicts the mechanisms by which SNAP-25 contributes to postsynaptic function. SNAP-25 has a role in the removal of KARs [8] and in the insertion of NMDA receptors in neuronal plasma membrane [7] , both processes involving PKC. Furthermore, through the interaction with p140Cap, SNAP-25 may stabilize a postsynaptic complex including cortactin [13] , Arp2,3, actin and actin capping proteins [51] , [60] , thus having a role in spine morphogenesis. Full size image Dendritic spines are small neuronal protrusions that regulate synaptic strength. Spines can be classified in three main types: filopodia-like protrusions (the more immature kind of spines), stubby spines that do not present a well-defined neck and mushroom spines (the mature dendritic spines) that are characterized by a large bulbous head and a constricted neck [39] . Hippocampal neurons present thousands of these spines on their dendrites [40] . In this study, we describe a post-synaptic role for SNAP-25 in modulating spine morphology and function. In particular, we show that reduction of SNAP-25 expression leads to a morphologically immature phenotype of dendritic spines that are, consistently, less functional. Over-expression of SNAP-25 results instead in an increase in the density of mushroom spines as well as of PSD95 puncta. The localization of SNAP-25 at the plasma membrane is essential for the protein role in controlling spine morphogenesis, thus suggesting that the protein acts as a scaffold protein that brings and/or retains other interactors to the membrane. Consistently, we demonstrate that SNAP-25 acts on spine morphology through the adaptor protein p140Cap [10] , [37] , a key protein involved in the regulation of spine morphogenesis [13] . SNAP-25 has a crucial role at the presynaptic level, where it mediates synaptic vesicles fusion [3] , [41] , [42] , [43] . Despite its key presynaptic function, the protein lacks a selective presynaptic distribution, being instead more diffusely localized throughout the neuronal plasma membrane [34] . Notably, a previous proteomic study demonstrated that SNAP-25 co-purifies with PSD-95 [44] . Although not univocally excluding that the presence of SNAP-25 in the PSD structure could be due to contamination from the pre-synapse, these data hint at a plausible post-synaptic localization for the protein. In line with being present also at the somatodendritic level, SNAP-25 controls calcium dynamics in the soma of cultured neurons [29] , [45] . In addition, SNAP-25 co-immunoprecipitates with the KAR subunits GluK5 and has a role in the removal of KARs from the postsynaptic membrane [8] . SNAP-25 phosphorylation by Protein Kinase C (PKC) is of fundamental importance for the insertion of NMDA receptors in neuronal plasma membrane [7] . In line with the SNARE role in postsynaptic function, amplitude of mEPSCs was reported to be reduced in the absence of SNAP-25 [46] , [47] , while exogenous expression of either SNAP-25a or SNAP-25b rescued the amplitude value [47] . Finally, a recent report showed that downregulation of the protein impairs potentiation phenomena [48] . By three-dimensional (3D) reconstruction, virtual slicing of dendritic spines in low-density cultures and GSD, which allows protein localization with a precision of up to 20 nm, we show that SNAP-25 immunoreactivity can be occasionally detected, although it is not specifically enriched, in dendritic protrusions of cultured hippocampal neurons. Our results are in line with the possibility that SNAP-25, present at the plasma membrane of nascent dendritic spines, favors p140Cap relocalization at a site where, in the presence of the appropriate molecular milieu necessary for spine formation, the process of spine morphogenesis may start. Interestingly, while lower mEPSC frequency and amplitude were recorded upon reduction of SNAP-25 expression, a significant reduction of mEPSC frequency but not amplitude occurred in neurons in which p140Cap was downregulated. These data suggest that while reduced SNAP-25 levels impact both synaptic number and function, downregulation of p140Cap decreases the number of synapses without having major changes in the function or maturational state of the remaining ones, as already described for other postsynaptic proteins [49] , [50] . Conversely, the lack of changes in mEPCS frequency or amplitude recorded upon either SNAP-25 or p140Cap over-expression suggests that the morphogenetic role of the two proteins may be not accompanied, at least under acute over-expression conditions, by functional effects. SNAP-25/p140Cap may converge on different pathways to regulate spine morphology. p140Cap, which binds to the plus end of dynamic microtubules [13] , could promote the local reorganization of spines controlling the levels of active RhoA by decreasing Src-dependent tyrosine phosphorylation of the RhoA-specific GTPase activating protein p190RhoGAP. Through inhibiting the activity of Src kinases at dendritic spines, p140Cap may reduce the phosphorylation of critical substrates such as Cortactin [13] . Cortactin is a protein that is able to stabilize branched actin filament network in spines, thus leading to the formation of mature mushroom spines. Notably, cortactin activates the Actin-related protein 2/3 (Arp2/3) complex, which controls the nucleation of new actin filaments, thus allowing the formation of a branched cytoskeletal network, which is necessary for spine head enlargement (reviewed by Menna et al . [51] , Fig. 7d ). In the absence of SNAP-25, the higher mobility of p140Cap, detected by FRAP experiments, may impair p140Cap ability to organize the molecular apparatus needed for the formation of the spine. This impairment might impact the occurrence of downstream events, including inhibition of Src kinase activity, which is known to lead to spine formation [13] . The possibility that p140Cap controls spine head growth through Src kinase activity and regulation of cortactin and Arp2/3 complex is worthy of further investigation. It is however expected that, besides SNAP-25, additional proteins may cooperate to the local recruitment of the spine complex or compensate for it in the chronic absence of SNAP-25. Changes in spine morphology and number have a fundamental role in cognitive functions and, indeed, several neurological disorders such as autism spectrum disorders, schizophrenia and Alzheimer’s disease are linked to aberrant shape and number of dendritic spines [52] . SNAP-25 has been associated with psychiatric diseases such as attention deficit hyperactivity disorder, bipolar disorder and schizophrenia [24] , [25] , [36] . In addition to the role of SNAP-25 in these disorders, a decrease in SNAP-25 levels in mice deficient for the synaptic vesicle protein cysteine-string protein-α (CSPα) causes a massive neurodegeneration [28] . Our results open therefore the possibility that SNAP-25 can have a role in these synaptopathies not only by virtue of its presynaptic function, but also by directly acting at the post-synaptic level and controlling formation and maintenance of proper spine number and morphology. Further investigations in mice models displaying reduced SNAP-25 levels will clarify this point. Ethics statement All the experimental procedures followed the guidelines established by the Italian Council on Animal Care and were approved by the Italian Government decree No. 27/2010. Cell cultures Rat hippocampal neurons were established from the hippocampi of embryonic stage E18 foetal rats. The dissociated cells were plated onto glass coverslips coated with poly- L -lysine at densities of 95 cells per mm 2 . The cells were maintained in Neurobasal medium (Invitrogen) with B27 supplement and antibiotics, 2 mM glutamine, and glutamate (neuronal medium). Plasmids SNAP-25Δ 86–120 construct was generated as follows: the sequence coding for first 84 aa with primer forward 5′-ATAAGAATGCGGCCGCATGGCCGAGGACGCAGAC-3′ containing the Not 1 restriction site, and reverse 5′-TTTGACGGACCTAGGAAAATTCGAATTCCG-3′ containing the Eco r1 site. The second fragment starting from the 121 aa until GFP tag at the C terminus of protein, was generated by amplification with primer forward 5′-CGGAATTCGTGGATGAACGGGAGCAGA-3′ containing the Eco r1 site, and reverse primer 5′-CAAATAATAAGGATCCAGATCTGCTG-3′ containing Bam HI site. After digestion, the two fragments were inserted into modified p-EGFPN1 vector cut with Not 1 and Bam HI. SNAP-25Δ 1–41 was generated by cloning into the modified p-EGFPN1 vector the fragments amplified from mouse SNAP-25 cDNA with the following primers: forward 5′-ATAAGAATGCGGCCGCATGGCTGGCATCAGGACTTTG-3′ and reverse 5′-CAAATAATAAGGATCCAGATCTGCTG-3′. p140Cap-GFP tagged construct was obtained as in the study by Di Stefano et al . [10] SNAP-25-GFP tagged construct was obtained as in the study by Verderio et al . [29] . p140CapΔ 649–696 construct was generated as follows: the first fragment coding 1–672 aa was obtained digesting the mouse p140Cap cDNA in p-EGFPN3 with Hin dIII and Sfb 1. The second coding 730- to the end of p140Cap was obtained by digesting mouse p140Cap cDNA in p-EGFPN3 with Sph 1 and Sal 1. The two fragments were cloned into p-EGFPN3 vector. SNAP-25Δ 181–206 and SNAP-25Δ 198–206 HA-tagged construct were obtained as in the study by Verderio et al . [29] . p140Cap-Cterm GFP was generated by cloning human p140Cap cDNA [10] into GFP-tagged pGW1. Acute downregulation of SNAP-25 and p140Cap expression Silencing of SNAP-25 was achieved via transfection of a pSUPER construct [29] . A nonspecific siRNA duplex of the same nucleotides, but in an irregular sequence (scrambled iSNAP-25 siRNA), was prepared using oligonucleotides 5′-GATCCCCGAGGAGTTATGCGATAGTATTCAAGAGAATGATAGCGTATTGAGGAGTTTTTGGAAA-3′ and 5′-AGCTTTTCCAAAAACTCCTCAATACGCTATCATTCTCTTGAATACTATCGCATAACTCCTCGGG-3′ that were annealed and ligated into the pSuper vector as described previously [29] . Silencing of p140Cap was achieved via transfection of a pSUPER construct. p140Cap-shRNA sequence (5′-CAGCCGAAACAGACTTCAG-3′) targeting rat p140Cap mRNA (nucleotides 2,771–2,789) was designed based on the experimentally verified human p140Cap-shRNA sequence [37] . The complementary oligonucleotides were annealed and inserted into pSuper vector [53] . Transfection Neurons were transfected using Lipofectamine 2000 (Invitrogen) at DIV 17–18. Cultures were analysed at DIV 20–21. Dendritic spines analysis Images of primary hippocampal cultures were acquired with a × 63 oil immersion lens (1,024 × 1,024 pixels). Each image consisted of a stack of images taken through the z -plane of the cell. Confocal microscope settings were kept the same for all scans in each experiment. For spine size, the maximal length was measured with the ImageJ software programme by manually drawing a vertical line from the base of the neck to the furthest point on the spine head. On the basis of morphology, spines were classified into the following categories: (1) Thin: spines with a long neck and a visible small head; (2) Mushroom: big spines with a well-defined neck and a very voluminous head; and (3) Stubby: very short spines without a distinguishable neck and stubby appearance [54] , [55] , [56] . Colocalization analysis Images of Hela cells were acquired with a × 63 oil immersion lens (1,024 × 1,024 pixels). Colocalization analysis was performed using Imaris analysis software. For the analysis, Manders’ colocalization coefficient was used. This coefficient has the advantage of providing two components: the fraction of A with B and the fraction of B with A. This is quite relevant for our analysis given that our probes distribute to different kinds of cellular components. Immunocytochemical staining Immunofluorescence staining [57] was carried out using the following antibodies: SNAP-25 (1:1,000; monoclonal, Sternberger Monoclonals), PSD95 (1:400; monoclonal; UC Davis/NIH NeuroMab Facility), p140Cap plyclonal antibody was generated as in the study by Di Stefano et al . [10] , Phalloidin (1:250, Alexa Fluor Phalloidin 555, Invitrogen). The counterstaining of nuclei was performed with DAPI (Sigma-Aldrich). Images were acquired using a Leica SPE confocal microscope. Co-immunoprecipitation Brain tissues were frozen in liquid nitrogen. Brain proteins were extracted with lysis buffer (1% NP40, 150 mM sodium chloride, 50 mM Tris–HCl, pH 7.5, 5% glycerol, 1 mM MgCl 2 , protease inhibitors (Roche, Basel, Switzerland) and 1 mM phenylmethylsulphonyl fluoride, 1 mM Na 3 VO 4 , 1 mM NaF, 1 mM DTT). For immunoprecipitation assays, 5 mg of total extract were precleared and incubated overnight at 4 °C with 1 μg of crosslinked antibody per mg of total protein. IPs were washed five times with lysis buffer. IPs and 50 μg of total brain extract were resolved by reducing SDS–PAGE and transferred to PVDF filters, which were incubated with the indicated antibodies and developed by using the ECL system. The following antibodies were used: p140Cap plyclonal antibody was generated as in the study by Di Stefano et al . [10] , HSP90 (1:1,000, monoclonal; BD Bioscience), SNAP-25 (1:1,000, monoclonal; Chemicon), PSD-95 (1:4,000, monoclonal; UC Davis/NIH NeuroMab Facility). GST: homemade monoclonal antibody was raised against Glutathione S-transferase protein. Antibodies crosslinking was performed as described in the study by Meixner et al . [58] . Electrophysiology Whole-cell patch-clamp recordings of miniature EPSCs were obtained from 20–21 DIV transfected hippocampal-cultured neurons. During recordings, cells were bathed in an external solution containing (in mM): 125 NaCl, 5 KCl, 1.2 MgSO 4 , 1.2 KH 2 PO 4 , 2 CaCl 2 , 6 glucose, and 25 HEPES-NaOH, pH 7.4. Tetrodotoxin l μM, Bicuculline 20 μM and AP5 50 μM (Tocris). Recording pipettes were filled with the intracellular solution containing (in mM): 130 K-gluconate, 10 KCl, 1 EGTA, 10 HEPES-NaOH, 2 MgCl 2 , 4 MgATP and 0.3 Tris-GTP. Recordings were performed at room temperature in voltage clamp mode at holding potential of −70 mV using a Multiclamp 700B amplifier (Molecular Devices) and pClamp-10 software (Axon Instruments, Foster City, CA, USA). Series resistance ranged from 10 to 20 MΩ and was monitored for consistency during recordings. Cells in culture with leak currents >100 pA were excluded from the analysis. Signals were amplified, sampled at 10 kHz, filtered to 2 or 3 KHz, and analysed using pClamp-10. GSD microscopy GSD was performed on a Leica SR GSD system. Samples were fixed and stained [57] . GSD is a super-resolution technique that allows single-molecule localization. The collection of overlapping fluorophores in the diffraction-limited image is separated to permit the detection of single dyes. This allows building a high-resolution image. In order to achieve GSD, high-power lasers are used to transfer fluorophores into long-lived dark states, a non-fluorescent molecule state. As soon as single fluorophores return from the dark state, new photons are recorded and localized by the system. This process is stochastic. The positions of these signals are then used by the software to reconstruct a super-resolution image with a precision up to 20 nm. Preparation of PSD fractions To isolate PSDs from rat hippocampus, a modification of the method of Gardoni et al . [59] was used. Animals were killed and hippocampi (from 15 animals) were rapidly dissected and pooled. Homogenization was carried out in a Teflon glass homogenizer (700 r.p.m.) in 4 ml g −1 of cold 0.32 M sucrose containing 1 mM HEPES, 1 mM MgCl 2 , 1 mM NaHCO 3 and 0.1 mM phenylmethylsulfonyl fluoride (pH 7.4) in the presence of complete sets of protease and phosphatase inhibitors. The homogenized tissue was centrifuged at 1,000 g for 10 min. The resulting supernatant was centrifuged at 3,000 g for 15 min to obtain a P2-crude membrane fraction. The P2 pellet was resuspended in 2.4 ml g −1 of 0.32 M sucrose containing 1 mM HEPES, 1 mM NaHCO 3 and 0.1 mM phenylmethylsulfonyl fluoride, overlaid on a sucrose gradient (0.85–1.0–1.2 M), and centrifuged at 82,500 g for 2 h. The synaptosomal fraction (Syn) between 1.0 and 1.2 M sucrose was removed, diluted with an equal volume of 1% Triton X-100 in 0.32 M sucrose containing 1 mM HEPES and incubated for 15 min. This solution was then spun down at 82,500 g for 30 min. The pellet (triton-insoluble fraction) was resuspended, layered on a sucrose gradient (1.0–1.5–2.1 M), and centrifuged at 100,000 g at 4 °C for 2 h. The fraction between 1.5 and 2.1 M was removed and diluted with an equal volume of 1% Triton X-100 and 150 mM KCl. PSDs were collected by centrifugation at 100,000 g at 4 °C for 30 min and stored at −80 °C. Protein content of the samples has been quantified by using Bio-Rad (Hercules, CA, USA) protein assay. Fifteen micrograms per sample were loaded in each lane. Western blot analysis was performed by using the following antibodies: PSD-95 (1:3,000, monoclonal; Neuromab), synaptophysin (1:3,000, monoclonal, Sigma-Aldrich), SNAP-25 (1:150,000; monoclonal, Sternberger Monoclonals), SNAP-25 (1:1,000, monoclonal; Chemicon), SNAP-25 (1:10,000, polyclonal; Synaptic Systems). p140Cap polyclonal antibody was generated as in the study by Di Stefano et al . [10] , alpha1A (1:500, polyclonal, Sigma-Aldrich), syntaxin 1 (1:1,000, monoclonal, Sigma-Aldrich). Western blotting was performed by means of Chemi-Doc system+Image Lab software (Bio-Rad). Fluorescence Recovery After Photobleaching FRAP experiments were performed as in the study by Jaworski et al . [13] using a FV1000-IX91 confocal microscope from Olympus. The 488-nm laser line was used for bleaching. Areas including the bleached spine were selected and the background was subtracted frame-by-frame by subtracting the average intensity of a not bleached area. Recovery was calculated using this formula: R =( I ( t )−I (directly after bleaching))/( I (before bleaching)−I (directly after bleaching). I=total spine intensity, R=recovery. R final =the level at the end of the recording (590 s after bleaching). Immobile fraction=1−R final . How to cite this article: Tomasoni, R. et al . Snap-25 regulates spine formation through postsynaptic binding to p140cap. Nat. Commun. 4:2136 doi: 10.1038/ncomms3136 (2013).